Linking experiment and theory for three-dimensional networked binary metal nanoparticle–triblock terpolymer superstructures Controlling superstructure of binary nanoparticle mixtures in three dimensions from self-assembly opens enormous opportunities for the design of materials with unique properties. Here we report on how the intimate coupling of synthesis, in-depth electron tomographic characterization and theory enables exquisite control of superstructure in highly ordered porous three-dimensional continuous networks from single and binary mixtures of metal nanoparticles with a triblock terpolymer. Poly(isoprene- block -styrene- block -( N,N -dimethylamino)ethyl methacrylate) is synthesized and used as structure-directing agent for ligand-stabilized platinum and gold nanoparticles. Quantitative analysis provides insights into short- and long-range nanoparticle–nanoparticle correlations, and local and global contributions to structural chirality in the networks. Results provide synthesis criteria for next-generation mesoporous network superstructures from binary nanoparticle mixtures for potential applications in areas including catalysis. Controlling the spatial arrangement of metal and semiconductor nanoparticles (NPs) from bottom-up self-assembly remains a long-standing scientific goal in materials synthesis [1] , [2] , [3] , [4] , [5] , [6] , [7] , [8] , [9] , [10] . Assembly of NPs as artificial ‘atoms’ into ordered structures provides facile access to a variety of previously unknown nanomaterials. Effective control over electrostatic and entropic interactions between NPs leads to highly ordered materials with structural diversity [2] , [3] , [4] , [5] , [9] . Complementary molecules, for example, DNA [1] , [9] , [10] or block copolymers (BCPs) [11] , attached to NPs mediate their ordered assemblies enabling programmable structure control. Despite this progress, major challenges remain in controlling the structures of metal and semiconductor NP assemblies at the mesoscale—for example, to provide mesoporosity as well as three-dimensional (3D) connectivity, highly desirable for applications requiring efficient charge transport in electrodes or electrocatalytic materials [12] , [13] , [14] . In particular, highly ordered mesoporous 3D bicontinuous network superstructures of metal NPs have stayed elusive, especially from mixtures of different NPs. Such 3D network structures, particularly if they are mesoporous, are of specific interest as they are expected to provide excellent mechanical stability, high accessibility to NP surface area and high connectivity. Here, we demonstrate how the combination of controlled NP synthesis, detailed structural analysis by transmission electron microtomography (TEMT) [15] , energy-dispersive X-ray spectroscopy (EDS) and percolation theory, as well as comparison with a recently developed self-consistent field theory (SCFT) [16] , [17] enabled highly ordered and porous 3D network formation of single and binary metal NPs from triblock terpolymer self-assembly with particle locations that can be rationalized. Analysis further provided insights into short- and long-range NP–NP correlations, and local and global contributions to structural chirality in an alternating gyroid (G A ) domain. Alternating gyroid structure Gyroid structures have been observed in low molar mass surfactant-water systems and BCP self-assembly [18] , [19] based on the minimal gyroid surface (Schoen’s G-surface, symmetry ) [20] . Structures in these systems usually consist of two intertwining gyroid subvolumes related by an inversion operation. If these two subvolumes are constituted by the same material, the structure is a double gyroid (G D , ). Each gyroid network contains chiral helices along various crystallographic directions. In the G D local chirality is cancelled, since respective screw axes of each gyroid network are of opposite handedness. The alternating (single) gyroid (G A , /4 1 32), in contrast, contains two subvolumes of different materials, thus exhibiting local chirality. The G A structure is found in several tropical butterfly species and depicts a unique chiral 3D periodic morphology [21] . While the periodic G D network structure is accessible via di-BCP self-assembly, the G A structure is only accessible via triblock terpolymers, which provides three distinct periodic block volumes. Triply periodic network phases formed by triblock terpolymers also form over much wider composition windows (4–14 vol%) [22] , [23] than the G D structure found in di-BCPs (2–6 vol%) [24] , [25] . Furthermore, mesoporous materials derived from the G A phase typically have larger pore volume than those from the G D phase. Finally, we also note that the chiral nature of the G A structure can lead to interesting properties [26] . Synthesis of terpolymer and hybrids Precise control of spatial organization of ligand-stabilized platinum (Pt) and gold (Au) NPs was achieved with a novel triblock terpolymer, poly(isoprene- block -styrene- block -( N,N -dimethylamino)ethyl methacrylate) (PI- b -PS- b -PDMAEMA), which will be referred to as ISA, ( Fig. 1a–c ). Polymer ISA had a molar mass of 102,300 g mol −1 , a poydispersity index below 1.1, and a composition of I, S and A of 23.4, 71.5 and 5.1 wt%, respectively (see Methods and Supplementary Fig. 1a ). Ligand-stabilized Pt NPs were synthesized by an improved synthesis scheme, while Au NPs were prepared according to known methods; see Methods. Ar-O plasma etching of organics resulted in 3D mesoporous metal networks comprising one or two different types of metal NPs. 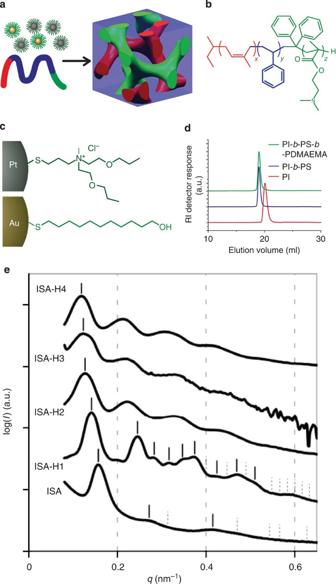Figure 1: Hybrid synthesis components and schematic as well as characterization results. (a) Scheme of triblock terpolymer–binary Pt and Au NPs self-assembly; (b) molecular structure of PI-b-PS-b-PDMAEMA (ISA); (c) molecular structure of ligands attached to Pt,N,N-di-(2-(allyloxy)ethyl)-N-3-mercaptopropyl-N-methylammonium chloride and Au NPs, 11-mercapto-1-undecanol; (d) size exclusion chromatograph data for different triblock terpolymer synthesis steps; (e) from bottom to top SAXS data of neat polymer ISA, Pt NP hybrid ISA-H1, binary Pt and Au NP hybrids ISA-H2, ISA-H3 and ISA-H4 with increasing Au NP content. Tick marks show expected peak positions for hexagonal (ISA) and GA(ISA-H1) structures. Solid and dotted tick marks distinguish between observed and missing peaks for ISA and ISA-H1, respectively. The tick mark positions for ISA-H2, ISA-H3 and ISA-H4 are used for determining the lattice spacingainTable 1. Figure 1: Hybrid synthesis components and schematic as well as characterization results. ( a ) Scheme of triblock terpolymer–binary Pt and Au NPs self-assembly; ( b ) molecular structure of PI- b -PS- b -PDMAEMA (ISA); ( c ) molecular structure of ligands attached to Pt, N,N -di-(2-(allyloxy)ethyl)- N -3-mercaptopropyl- N -methylammonium chloride and Au NPs, 11-mercapto-1-undecanol; ( d ) size exclusion chromatograph data for different triblock terpolymer synthesis steps; ( e ) from bottom to top SAXS data of neat polymer ISA, Pt NP hybrid ISA-H1, binary Pt and Au NP hybrids ISA-H2, ISA-H3 and ISA-H4 with increasing Au NP content. Tick marks show expected peak positions for hexagonal (ISA) and G A (ISA-H1) structures. Solid and dotted tick marks distinguish between observed and missing peaks for ISA and ISA-H1, respectively. The tick mark positions for ISA-H2, ISA-H3 and ISA-H4 are used for determining the lattice spacing a in Table 1 . Full size image SAXS characterization of hybrid films With the synthesis of the ISA triblock terpolymer and careful choice of the NP ligands, we obtained networked hybrid materials with Pt metal NPs as well as with binary mixtures of Pt and Au metal NPs (see Table 1 for hybrid compositions). We first characterized the NP superstructures by small-angle X-ray scattering (SAXS). Figure 1e compares SAXS results of the parent ISA and the resulting hybrids obtained by polymer NP mixing in a common solvent and subsequent casting of films (see Methods). Neat ISA showed a microphase-separated hexagonal morphology as suggested by SAXS and transmission electron microscopy (TEM; Fig. 1e and Supplementary Fig. 1b ). Table 1 Terpolymer–binary metal NP hybrid compositions. Full size table Hybrid ISA-H1 with 23.1 wt% Pt NPs exhibited a scattering curve containing up to 10 higher-order peaks, very different from the parent polymer trace. Tick marks in Fig. 1e for this scaling trace show expected peak positions for a G A lattice with I 4 1 32 space group, with ( q/q 100 ) 2 =2, 6, 8, 10, 12, 14, 16, 18, 20, 22, 24, 26, 30, 32, 34, where the scattering vector q is defined by q =4 π sin θ / λ , with scattering angle 2 θ , X-ray wavelength λ and reciprocal vector, q 100 , describing the cubic lattice parameter. Expected and observed peak positions match well, suggesting that the SAXS trace of the hybrid is consistent with the G A morphology. The narrow first-order peak and clear higher-order peaks further suggest well-defined interfaces and large grain sizes. Addition of Pt NPs to ISA thus resulted in a phase transformation from a hexagonal to a cubic network (G A ) structure. We further increased the loading of Pt NPs resulting in lamellar morphology as predicted from theory [17] (see Supplementary Fig. 1c for the morphology map of ISA-Pt NP hybrids). TEM characterization of hybrid films The assignment of hybrid morphology was corroborated by TEM characterization. 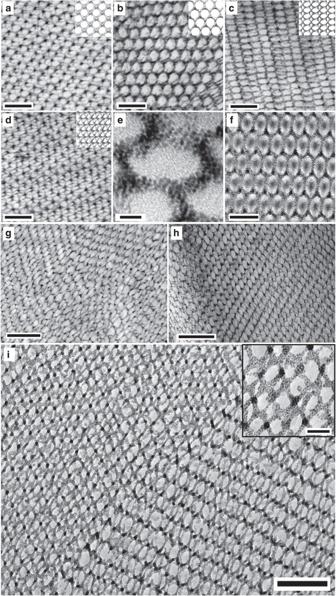Figure 2: TEM characterization of materials. Representative TEM images of ISA-H1 (a–f), ISA-H2 (g) and ISA-H3 (h) before removal of organic materials. ISA-H1 film with about 100 nm thickness was further treated with Ar-O plasma for 20 min and its TEM image is shown ini. (a–f) ISA-H1 with different projections: (a), (100); (b), (111); (c), (110); (d), (210); (e), higher magnification image showing individual Pt NPs; (f), (111) projection with PI domain stained by OsO4. Insets show SCFT simulations of expected contrast distributions for different projections; hybrids with binary Pt and Au NP mixtures, (g) ISA-H2 and (h) ISA-H3. (i) ISA-H1 after Ar-O plasma treatment at different magnifications (inset). Scale bars, 100 nm (a–d), 10 nm (e), 50 nm (f), 200 nm (g,h), 100 nm (i), 20 nm (inset ofi). Figure 2a–f shows representative TEM images of 100-nm-thick microtomed sections of hybrid ISA-H1 exhibiting different projections. The metal NP+PDMAEMA domains appear dark providing image contrast to the PI and PS domains. Fourfold (100) and threefold (111) projections ( Fig. 2a,b ) characteristic for a cubic structure can clearly be identified. Other planes, for example (110) and (210) planes, are also often observed in TEM, see Fig. 2c,d . Insets in Fig. 2a–d represent NP network images of the respective G A projection obtained from SCFT simulations, which match well with the experimental data. Quantitative analysis of TEM images stays challenging, however, as information of a 3D structure is reduced to a two-dimensional (2D) plane and because of possible PI domain distortions in microtomed thin slices originating from the low T g of PI (−60 °C). Indeed, the cubic lattice parameters, a , calculated from these images are all between 50 and 60 nm, that is, slightly underestimating the value of 63 nm from SAXS. Higher magnification TEM images of ISA-H1 ( Fig. 2e ) resolve individual Pt NPs filling the struts of the network structure. Staining PI domains with OsO 4 provided additional contrast to the material and enabled simultaneous visualization of struts of the two gyroid minority networks. Figure 2f shows the TEM image of a (111) projection of ISA-H1 where PI domains appear in light grey and Pt NP+PDMAEMA domains in dark. The image clearly reveals that the two domains form two networks that are intertwining with each other. Figure 2b,f also shows the triple node connectivity of the material, which is characteristic of gyroidal structures. Figure 2: TEM characterization of materials. Representative TEM images of ISA-H1 ( a – f ), ISA-H2 ( g ) and ISA-H3 ( h ) before removal of organic materials. ISA-H1 film with about 100 nm thickness was further treated with Ar-O plasma for 20 min and its TEM image is shown in i . ( a – f ) ISA-H1 with different projections: ( a ), (100); ( b ), (111); ( c ), (110); ( d ), (210); ( e ), higher magnification image showing individual Pt NPs; ( f ), (111) projection with PI domain stained by OsO 4 . Insets show SCFT simulations of expected contrast distributions for different projections; hybrids with binary Pt and Au NP mixtures, ( g ) ISA-H2 and ( h ) ISA-H3. ( i ) ISA-H1 after Ar-O plasma treatment at different magnifications (inset). Scale bars, 100 nm ( a – d ), 10 nm ( e ), 50 nm ( f ), 200 nm ( g , h ), 100 nm ( i ), 20 nm (inset of i ). Full size image Mesoporous film formation To maintain the superstructure on removal of the structure-directing polymer on the way to mesoporous materials, NP percolation in all three directions is needed. A percolation analysis shows that ISA-H1 is very close to a NP percolation threshold [27] suggesting that the superstructure may survive ISA removal (see ‘NP percolation’ paragraph in Methods section and Supplementary Fig. 2 ). Ar-O plasma treatment of 100 nm slices of as-made hybrids was used to test this hypothesis. The high quality structure control in the resulting porous NP superstructures is revealed in the representative TEM image of sample ISA-H1 in Fig. 2i showing the boundary between two grains running diagonally through the middle of the image. The individual Pt NPs constituting the superstructure can clearly be distinguished in the higher magnification image in the inset of Fig. 2i . EDS data indicate that a large fraction of organic materials including the ligands were etched away during the plasma treatment; see Supplementary Fig. 3 . However, because of the low X-ray fluorescence yield of carbon atoms, quantification of organic content after plasma treatment has a rather large error bar associated with it. From the spectra in Supplementary Fig. 3c alone, it is thus not possible to exclude remaining organic material. The porous NP superstructure survived the plasma treatment probably because of NP percolation mediated by shrinkage of the gyroidal network while removing organic materials (see ‘NP percolation’ paragraph in Methods section). 3D local, global and chiral structures characterization A 3D TEMT reconstruction provides visualization of the 3D nanostructure in real space at a resolution of a few Angstroms, high enough to distinguish individual NPs [15] . Reconstruction of the 3D superstructure of as-made hybrid ISA-H1, that is, without the plasma treatment, was chosen for G A structure analysis owing to the best long-range order among all hybrids. Results are shown in Fig. 3 where red spheres represent the Pt NP cores. Since NPs are coated with ligands, most of the NP cores are separated (note that identification of organic parts of the hybrid, that is, polymers and ligands, is challenging because of their small electron density contrast; see also Fig. 2 ). From reconstruction of NP cores the 3D superstructure is not easily identified. This could be achieved by increasing the NP diameters, that is, by convoluting the NP cores with a sphere of diameter d . The resulting overlapping volumes for the case of d= 6.5 nm are shown via the green surfaces in Fig. 3 , clearly giving rise to a simple network structure. To further demonstrate that this network is consistent with the G A morphology, we compared it with a superimposed G A network obtained from a SCFT simulation; see the bottom right of Fig. 3 . 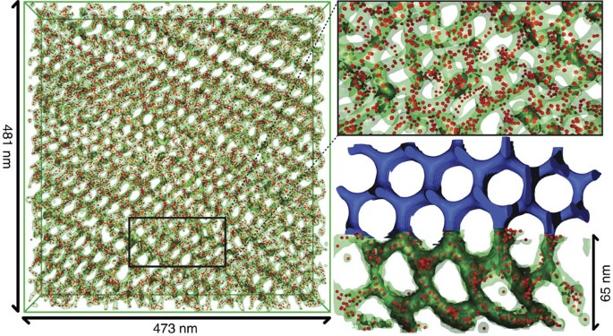Figure 3: TEMT reconstruction of Pt NP network superstructure in as-made ISA-H1 and comparison with SCFT results. The sample was imaged without the plasma treatment. Red spheres are Pt NPs and green volumes represent networks formed by enlarging the radii of NP cores. On the lower right a blue gyroid network with (111) projection obtained by a SCFT approach is superimposed for comparison. Figure 3: TEMT reconstruction of Pt NP network superstructure in as-made ISA-H1 and comparison with SCFT results. The sample was imaged without the plasma treatment. Red spheres are Pt NPs and green volumes represent networks formed by enlarging the radii of NP cores. On the lower right a blue gyroid network with (111) projection obtained by a SCFT approach is superimposed for comparison. Full size image Chirality of G A morphology is intriguing since all of the molecules in the self-assembly system are achiral (see Fig. 1b,c ). Therefore, a racemic mixture of chiral network domains is expected. We identified local and global chirality of ISA-H1 via structural simplification technique since 3D network structures are usually complex. Applying a surface-thinning algorithm to the reconstruction data [28] , [29] , we skeletonized the 3D networks and quantized NP network connectivity. Before application to experimental data, as an example we analysed a theoretical G A NP network obtained by the SCFT (see Fig. 4a ). As expected for the G A morphology [30] , triple nodes and struts are successfully identified in the cubic unit cell and defects are found only on the artificially cleaved surface planes. A similar situation is found for the reconstructed slab where defects are focused on the edges of the slab (see Fig. 4b ). However, a small number of defects can also be clearly identified within the reconstructed sample volume. 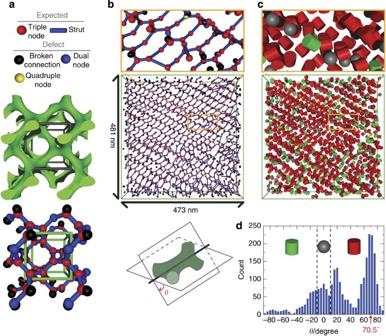Figure 4: Identification of local and global contributions to structural chirality in gyroidal networks of ISA-H1. (a) A 2 × 2 × 2 cubic unit cell of a chiral GANP network obtained from SCFT simulation (top); nodes and struts identified via a surface-thinning algorithm (bottom)28. The black and green boxes represent a cubic unit cell in the simulated and thinned structures, respectively. For the GAnetwork, triple nodes and struts can be identified, for example, inside of the green cubic unit cell30and defects are found only on artificially cleaved planes. (b) Network connectivity of NPs obtained by the surface-thinning algorithm, where NP core diameters are enlarged tod=6.5 nm (green networks inFig. 3) and the same colour codes as inaare used. Thin top and bottom layers, about one-sixth of the sample for each layer, are not shown because defects in the layers were generated during the thin hybrid sample preparation. (c) Chirality of each node is identified from rotation angles of neighbouring gyroidal node planes,θ; see model. Red cylinders correspond to clockwise (θ=10°~90°), green cylinders to counter-clockwise (θ=−10°~−90°) and grey spheres to other rotation angles (θ=−10°~10°). Cylinder axes represent directions normal to gyroidal node plane. (d) Histogram for experimental rotation angles. The largest population is observed at 70.5°, which is the theoretically expected value for gyroidal nodes. Figure 4: Identification of local and global contributions to structural chirality in gyroidal networks of ISA-H1. ( a ) A 2 × 2 × 2 cubic unit cell of a chiral G A NP network obtained from SCFT simulation (top); nodes and struts identified via a surface-thinning algorithm (bottom) [28] . The black and green boxes represent a cubic unit cell in the simulated and thinned structures, respectively. For the G A network, triple nodes and struts can be identified, for example, inside of the green cubic unit cell [30] and defects are found only on artificially cleaved planes. ( b ) Network connectivity of NPs obtained by the surface-thinning algorithm, where NP core diameters are enlarged to d= 6.5 nm (green networks in Fig. 3 ) and the same colour codes as in a are used. Thin top and bottom layers, about one-sixth of the sample for each layer, are not shown because defects in the layers were generated during the thin hybrid sample preparation. ( c ) Chirality of each node is identified from rotation angles of neighbouring gyroidal node planes, θ ; see model. Red cylinders correspond to clockwise ( θ =10°~90°), green cylinders to counter-clockwise ( θ= −10°~−90°) and grey spheres to other rotation angles ( θ =−10°~10°). Cylinder axes represent directions normal to gyroidal node plane. ( d ) Histogram for experimental rotation angles. The largest population is observed at 70.5°, which is the theoretically expected value for gyroidal nodes. Full size image The chirality of individual gyroidal nodes was identified by calculating the angle difference between planes of neighbouring triple nodes as shown in Fig. 4 (note that the networks with d= 6.5 nm, green networks in Fig. 3 , were used for identifying the chirality since the network connectivity barely changes above this value, see Supplementary Fig. 2 ). As the histogram in Fig. 4d shows, most gyroidal nodes have a clockwise rotation, that is, positive angle, and the largest population is at θ≈ 70.5°, which is the theoretically expected value for gyroidal nodes [22] . Since counter-clockwise rotations seem to come mostly from self-assembly defects as well as artificial defects from the thin sample preparation, the sample is effectively a single chiral domain. Point, line and plane defects are observed, while chiral domain boundaries are not identified in the 3D data set (see Fig. 4b,c ). Although only a submicron sample area was characterized, one can expect large (several tens of microns) chiral domain formation, as recently observed in the far-field optical characterization of BCP and electrodeposition-derived G A metamaterials [26] , where circularly polarized light propagation was observed as predicted for chiral domains [31] . Ligand density effect on nanoparticle superstructure Having established the local and global structural characteristics of the G A hybrid, for a better understanding of the underlying physics of this self-assembly system, we quantitatively compared the experimental results with predictions from a SCFT approach, a field theoretic approach that enables predictions of self-assembled materials morphology at the mesoscale, usually challenging for particle-based simulations [16] , [23] , [32] , [33] , [34] . To that end, we recently developed a theory that allowed study of ABC terpolymer/ligand-stabilized NP self-assembly and predicted G A NP network formation, where the C block had affinity to ligand-stabilized NPs thus corresponding to PDMAEMA in the current experiments [16] , [17] . For direct comparison, 2D NP distributions, projected along the (111) direction, were calculated for the 3D reconstruction data ( Fig. 5b ) and from results of two different SCFT simulations ( Fig. 5c,e ). As a reference system, one of the simulated systems in Hur et al. [17] was chosen; see results in Fig. 5b (see Methods section and Supplementary Fig. 4 for a more detailed description). A more dispersed NP distribution is observed in the reference system than in the experiment (compare Fig. 5b,c ). To better account for the true experimental structure of the ligand-stabilized NPs ( N L =60.8 and branched ligand), the number of ligands per NP was increased by a factor of 3, to N L =60, and ligands were made two times larger [35] . The resulting simulated NP density distribution in Fig. 5e is almost identical to the one found experimentally ( Fig. 5b ). 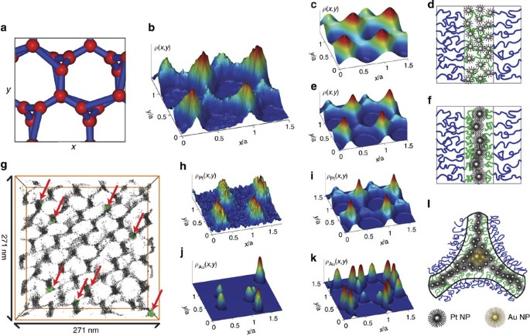Figure 5: Quantitative comparison of NP locations between experiment and theory. 3D data analyses of (b–f) single and (g–l) binary metal NP systems. NP distribution profiles projected along (111) direction,ρ(x,y), were compared between (b,h,j) experiments and (c,e,i,k) SCFT simulations: (a) (111) projection of gyroidal nodes (red spheres) and struts (blue cylinders) of GA; (b) Pt NPs of ISA-H1; (c) NPs of Huret al.17; (d) illustration of NP distribution ofcin a strut; (e) NPs with three times more (NL=60) and two times larger ligands than those inc; (f) illustration of NP distribution ofbandein a strut; (g) TEMT and EDS elemental mapping of Pt (black) and Au (green) NPs in the polymer-containing hybrid ISA-H4, where Au NPs are indicated by red arrows; (h) Pt NPs of ISA-H4; (i) Pt NPs of SCFT simulation; (j) Au NPs of ISA-H4; (k) Au NPs of SCFT simulation; and (l) illustration of NP distribution ofh–kin a gyroidal node. Note thatainb,c,eandh–kis the cubic lattice parameter. Figure 5: Quantitative comparison of NP locations between experiment and theory. 3D data analyses of ( b – f ) single and ( g – l ) binary metal NP systems. NP distribution profiles projected along (111) direction, ρ(x,y) , were compared between ( b , h , j ) experiments and ( c , e , i , k ) SCFT simulations: ( a ) (111) projection of gyroidal nodes (red spheres) and struts (blue cylinders) of G A ; ( b ) Pt NPs of ISA-H1; ( c ) NPs of Hur et al. [17] ; ( d ) illustration of NP distribution of c in a strut; ( e ) NPs with three times more ( N L =60) and two times larger ligands than those in c ; ( f ) illustration of NP distribution of b and e in a strut; ( g ) TEMT and EDS elemental mapping of Pt (black) and Au (green) NPs in the polymer-containing hybrid ISA-H4, where Au NPs are indicated by red arrows; ( h ) Pt NPs of ISA-H4; ( i ) Pt NPs of SCFT simulation; ( j ) Au NPs of ISA-H4; ( k ) Au NPs of SCFT simulation; and ( l ) illustration of NP distribution of h – k in a gyroidal node. Note that a in b , c , e and h – k is the cubic lattice parameter. Full size image Owing to a larger effective volume, NPs with more and larger ligands tend to be more aggregated to the centres of gyroidal triple nodes and struts (see Fig. 5a for structural details of gyroidal triple nodes and struts projected along (111) direction) similar to large NPs segregating to the middle of lamellae in a 1D lamellar morphology [34] . Entropic driving forces of mixing for larger molecular objects are weak. Thus, enthalpic driving forces dominate self-assembly and induce NPs to be more separated away from enthalpically repulsive blocks (see illustrations in Fig. 5d,f ). Other experimental factors have much weaker effects on NP distribution than the ligands (see Supplementary Fig. 4 ). The radial distribution function of Pt NPs as a function of NP to NP distance, r , in Fig. 6a , as obtained from analysis of the reconstruction data, details both short- and long-range NP–NP correlations. The maximum is observed at r≈ 3 nm, much smaller than the NP diameter (~5 nm) including the ligand layer (3–3.6 nm; note that the average NP core diameter is about 1.8 nm (ref. 35 )). This suggests that the majority of the NPs are interdigitated. Close inspection of the reconstruction data reveals that NP ligands are aggregated mostly in the triple nodes, while NPs in the struts are mostly disconnected. The SCFT simulation reveals the highly aggregated regime (triple nodes) and the sparse NP regime (struts) as shown in Fig. 6b . The aggregation in triple nodes is experimentally corroborated via long-range correlation peaks of the radial distribution function that coincide with distances from a node to a nearest neighbour ( r= 21 nm) and a second nearest-neighbour node ( r= 39 nm). This corresponds to a cubic lattice dimension of a= 59 nm, close to the value of 63 nm as measured by SAXS (see the inset of Fig. 6a ). 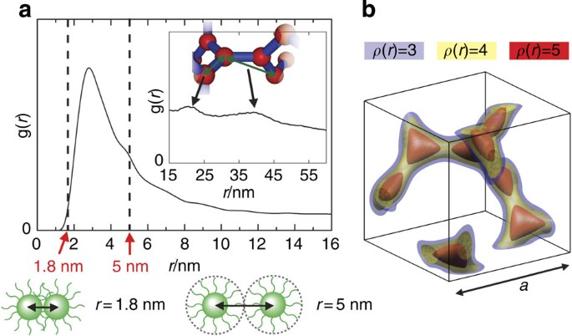Figure 6: Short- and long-range NP–NP correlations. (a) Radial distribution function,g(r), of NPs as a function of distance,r, from tomographic data set of ISA-H1. The inset details long-range correlations in the data. (b) Isosurfaces of NP density from the SCFT simulation ofFig. 4cat three different densities (a.u.). Highly concentrated NP distributions are observed in triple nodes, shown as red spheres in the inset ofa. The cubic lattice parameter,a=59 nm, based on distances from a node to a nearest neighbour (r=21 nm) and a second nearest-neighbour nodes (r=39 nm) is close to the value of 63 nm obtained from SAXS on the experimental system. Figure 6: Short- and long-range NP–NP correlations. ( a ) Radial distribution function, g(r) , of NPs as a function of distance, r , from tomographic data set of ISA-H1. The inset details long-range correlations in the data. ( b ) Isosurfaces of NP density from the SCFT simulation of Fig. 4c at three different densities (a.u.). Highly concentrated NP distributions are observed in triple nodes, shown as red spheres in the inset of a . The cubic lattice parameter, a= 59 nm, based on distances from a node to a nearest neighbour ( r= 21 nm) and a second nearest-neighbour nodes ( r= 39 nm) is close to the value of 63 nm obtained from SAXS on the experimental system. Full size image Control of binary metal NPs superstructure The ligand density on the Pt NP surface is a key parameter for governing spatial arrangement of the NPs in this self-assembly system. Moving a step further, we hypothesized that ligand chemistry may control the NP spatial arrangement in binary NP-based 3D network superstructures. The hypothesis was tested via synthesis of a metal NP with higher ligand density than observed for the Pt NPs. For controlled experiments, a newly synthesized NP should have similar NP metal core diameter but should be distinguishable from the Pt NP in an electron microscope. We achieved these requirements by choosing Au and a linear molecule as NP metal core and ligand, respectively. A linear ligand is expected to yield higher ligand density on NP surface as compared with a branched ligand because of less steric repulsion between the ligands (see Fig. 1c ). Resulting Au NPs had similar metal core diameters but a ligand density 3.5 times as high as for Pt NPs (see Supplementary Fig. 5 ). We prepared binary NP hybrids from 18 to 20 wt% Pt and Au NPs, with 5, 10 and 15.8 wt% of the total NPs being Au, referred to as ISA-H2, ISA-H3 and ISA-H4, respectively (see Table 1 ). With increasing Au NP content, broadening of SAXS peaks was observed, indicating a more disordered lattice, along with a systematic lattice parameter increase in Fig. 1e . On the basis of these SAXS traces alone, structure assignments were not possible. TEM micrographs in Fig. 2g,h clearly established metal NP-based single networks for both ISA-H2 and ISA-H3. Thus, while maintaining a 3D NP superstructure, binary metal NPs composition can be programmed. A combination of TEMT and EDS provided independent spatial distribution of Pt and Au NPs (see Fig. 5g,h,j and Supplementary Fig. 6 ). Owing to the loss of long-range order as evidenced by the SAXS measurements in Fig. 1e , NP distribution of the binary system projected along (111) direction is less clear than that of the Pt NP system (compare Fig. 5b with h ). Interestingly, Au NPs are strongly localized only in gyroidal nodes (see green spheres indicated by red arrows in Fig. 5g and NP distribution in Fig. 5j ). To account for this phenomenon, we performed SCFT simulations of binary ligand-stabilized NP systems, where we used N L =210 for Au NPs to match the experimental conditions. However, such unusual localization of Au NPs to gyroidal nodes was not initially observed in the SCFT simulation (see Supplementary Fig. 7 ). Simulations with strong enthalpic repulsions between B blocks (PS block in experiment) and Au NPs, where interaction parameter, χ B,Ligand N , was changed from 14.2 to 40, reproduced such behaviour (compare Fig. 5k with Supplementary Fig. 7b ). To minimize the enthalpic energy penalty, Au NPs more repulsive to the B blocks than Pt NPs dominantly occupy gyroidal triple nodes (see Supplementary Fig. 8 ). Strong enthalpic repulsions between PS blocks and Au NP ligands are readily expected owing to the terminal hydroxyl group of the Au NP ligand (see Fig. 1c ). As for the case of Pt NPs only, binary NP hybrids could be treated with Ar-O plasma, resulting in mesoporous materials (see Supplementary Fig. 9 ). These results suggest that NP ligands dominantly govern the BCP/NP self-assembly. Careful design of NP ligands in terms of ligand density and interactions between NPs and BCPs can enable programmable control of the NP spatial arrangement in such 3D self-assembly systems. Interestingly, a recent study on superstructure formation in semiconductor quantum dot self-assembly also elucidated that ligand density and molecular structure are the key parameters governing NP assembly despite very distinct molecular structures [36] . In summary, we presented the preparation and analysis of highly ordered 3D single-network superstructures of single and binary metal NPs from triblock terpolymer/NP self-assembly. Plasma etching of the hybrids, both with Pt NPs and with Pt and Au NPs, resulted in porous materials without the loss of NP superstructure. Structures were studied at an unprecedented level of detail utilizing a combination of TEMT, EDS, SCFT and percolation analysis to understand the underlying physics of self-assembled NP superstructure formation. Analysis of NP radial distribution elucidated significant NP ligand interdigitation as well as long-range correlations owing to clustering of NPs in gyroidal nodes. We demonstrated how application of surface-thinning algorithms to the tomographic data allows detailed analysis of local and global contributions to structural chirality of the G A network. Finally, we found that careful design of ligand structure in binary metal NP terpolymer assembly can enable programmable control of the NP spatial arrangement in 3D single-network superstructures owing to its dominant effects on NP distribution. We expect that results of this study will help guide future fabrication of porous NP-based network superstructures for applications ranging from high charge density electrodes to high surface area catalysis. Triblock terpolymer preparation PI- b -PS- b -PDMAEMA (ISA, Fig. 1b ) was synthesized via sequential anionic polymerization [37] . As far as we know, this is the first report on the synthesis and properties of this terpolymer. Aliquots of samples were taken after each polymerization step for analysis. Figure 1d shows the size exclusion chromatography results for PI, PI- b -PS and the final triblock terpolymer PI- b -PS- b -PDMAEMA, demonstrating well-controlled polymerizations with narrow molar mass distributions (poydispersity index<1.1) after each step. The accurate molar mass of the first PI block was determined by size exclusion chromatograph against a PI calibration, while the final triblock terpolymer composition and molar mass was calculated based on 1 H NMR integration (see Supplementary Fig. 1a ) and the accurate PI molar mass. The final terpolymer had molar mass of 102,300 g mol −1 and 23.4 wt% PI, 71.5 wt% PS and 5.1 wt% PDMAEMA. Nanoparticle synthesis The synthesis of the Au NPs stabilized by the ligand 11-mercapto-1-undecanol used in this study is detailed in Zheng et al. [38] Ligand-stabilized Pt NPs were synthesized by a synthesis scheme that is improved over what was described in our previous work [6] , [35] . PtCl 4 (0.78 g) were dissolved in 200 ml H 2 O/methanol (1/1 v/v) solvent mixture (solution A). Ligand (0.30 g), N,N -di-(2-(allyloxy)ethyl)- N -3-mercaptopropyl- N -methylammonium chloride and 0.86 g NaBH 4 were taken out from the glove box and dissolved in 10 g methanol (ligand solution B) and 15 g H 2 O (NaBH 4 solution C), respectively. Solutions B and C were subsequently added into solution A quickly (within 5 s) while stirring vigorously. The solution colour changed from black to dark brown within 5 min, indicating the formation of sub 3-nm NPs. The solution was further allowed to stir for 45 min, and then 50 ml methanol was added to dilute the solution and terminate the reaction. Methanol was rotary evaporated out and the solution was freeze dried on a vacuum line to remove excess water. The NPs were subsequently dissolved in chloroform and filtered through filter paper to remove salts formed in the synthesis. To remove residual free ligand, the particles were finally washed with a chloroform/ethyl ether mixture for four to five times. The final Pt NPs were a black powdery solid. Hybrid synthesis The hybrid films were prepared via evaporation-induced self-assembly of ISA, Pt NPs and Au NPs from a common solvent. The solid components were mixed in a ratio listed in Table 1 and were dissolved in 9:1 (wt) chloroform/methanol mixture so that the total solid concentration was 10 wt%. The solutions were poured in aluminium dishes and were heated to 50 °C on a hotplate under a hemispherical dome to slow down the evaporation. Finally, the films were heated in a vacuum oven at 130 °C to remove the solvents. The resulting films were sectioned with a Leica FC7 cryoultramicrotome to 100 nm for electron microscopy imaging. Conventional TEM Sectioned samples before and after two to four cycles of 5 min Ar-O plasma treatment (Fischione Model 1020) were used. TEM images were acquired in a Tecnai T12 Spirit microscope with a LaB 6 source and 120 kV acceleration voltage ( Fig. 2 ; Supplementary Fig. 9 ). Scanning TEM (STEM) images with EDS data for ISA-H1 before and after plasma treatment were obtained in a Tecnai F20 FE-STEM operated at 200 kV acceleration voltage ( Supplementary Fig. 3 ). TEMT and EDS TEM samples before plasma cleaning were used for TEMT. Before TEMT of ISA-H1, Au NPs (diameter: 5 nm) were placed on the supporting membrane of the TEM grid. TEMT was performed on an electron microscope operated at 200 kV (JEM-2200FS, JEOL Co., Ltd., Japan) and equipped with a slow-scan charge-coupled device camera (Gatan USC4000, Gatan Inc., USA). A series of projection images were taken from −70° to +70° at an angular interval of 1°. The tilt series of images were aligned by the fiducial marker method using the Au NPs as fiducial markers [39] . After the alignment, 3D images were reconstructed by the filtered back projection algorithm [15] . For TEMT and EDS of ISA-H4, the thin section was coated with carbon on the upper side. Au NPs with 5 nm diameter were deposited on the back side of the thin section. The specimen was tilted from −71° to 65° at 1° steps. The tilting series of TEM images were acquired on a JEM-2200FS operated at 200 kV. After TEMT observation, EDS measurement at same field of view was carried out on a JEM-ARM200F operated at 200 kV. The EDS mapping images at four fields of view were combined into one mapping image. SAXS experiments SAXS patterns of samples were obtained at Cornell High Energy Synchrotron Source G1 station with a beam energy of 9 keV as well as at a home-built Rigaku RU300 CuKα rotating anode beamline. The details of both SAXS beamline configurations are described elsewhere [40] . Acquired 2D patterns were azimuthally integrated around the beam centre to produce intensity versus scattering vector magnitude, q , defined as q =4 π sin θ / λ , where 2 θ is the total scattering angle and λ is the X-ray wavelength. Network connectivity identification NPs were identified from 3D TEMT data by setting a large threshold that exceeds signals of organic components. The binary data, where the regime occupied by NP cores is 1 and otherwise 0, were convoluted with a sphere to form networks. Using a surface-thinning algorithm [28] , coordinates and branching orders of gyroidal nodes as well as connectivity between the nodes were obtained. Nanoparticle percolation Since NPs are coated with ligands, most of the NP cores are separated as in Fig. 3 (note that the identification of organic parts of the hybrid, that is, polymers and ligands, is challenging owing to small electron density contrast between them as shown in Fig. 2a–e ). Therefore, 3D superstructures are not easily identified. To identify NP superstructure, we increased NP core diameters for NP cores to overlap, thus forming continuous networks, that is, convoluted NP cores with a sphere with diameter d . Since the size of the ligand molecule with a fully stretched configuration is about 1.5~1.8 nm ( Supplementary Fig. 4 ), with d= 3.2 nm for the ligand layer thickness exhibits NP networks connected by ligands. Each regime in different colours in the bottom panels of Supplementary Fig. 2 corresponds to a NP network domain where NPs are connected within the domain and disconnected with NPs outside the domain. Since many NPs are separated farther than d= 3.2 nm in Supplementary Fig. 2 , relatively small domains are observed. A slight increase of d from the ligand layer thickness leads to formation of big domains (see the bottom panel of Supplementary Fig. 2c ). Such network domain formation can be detailed by a percolation theory [27] . For applying percolation theory, a gyroidal network domain can be simplified as a set of nodes connected by struts as in Fig. 4a . The node-to-node percolation depends on either open or closed strut connections, where the open and closed strut connections correspond to discontinuous and continuous NPs through the strut, respectively. Finite size domains are formed below a percolation threshold ( Supplementary Fig. 2a,b ), while an infinitely large domain is formed above the threshold ( Supplementary Fig. 2c–f ). The gyroidal network confines positional freedom of NPs within PDMAEMA blocks with larger NPs having higher chances of being continuous within the strut. Therefore, the node-to-node percolation probability, α , is approximately the volume ratio of NPs to NPs plus PDMAEMA block and estimated to be α =0.65 for our hybrid. Utilizing the percolation theory [27] , we can estimate the percolation threshold α c =1 /(Z −1)=0.5, where Z is the coordination number that characterizes the number of neighbouring nodes with Z= 3 for the gyroidal triple node. Thus, our hybrid sample is above the threshold, α c =0.5. Despite a larger α than the threshold for the case of d= 3.2 nm corresponding to an extended ligand conformation, however, small domains are observed in Supplementary Fig. 2b , implying that a realistic α is close to, but smaller than, α c owing to inhomogenous NP distribution (see the change of network connectivity and domain size as d increases in Supplementary Fig. 2 ). Please note that the inhomogeneity is consistent with results of the radial distribution function of NPs and NP density distributions of SCFT simulations as shown in Fig. 6 . The domain size below the critical point is expected to be a few cubic unit cells, that is, ~50 nm, since the number of cubic unit cells per domain is approximately given by 1/[1 −(Z−1)α]/ 10 (ref. 41 ) and order of 1 for 0.9 <(Z− 1 )α< 0.99 in close proximity to the critical point (note that the factor 10 comes from 10 triple nodes existing in a gyroid cubic unit cell [30] ). At the molecular level, NP ligands are interdigitated in the triple node while NPs are disconnected within the strut. Interestingly, the Pt NP superstructure was maintained after plasma treatment of hybrid ISA-H1 (see Fig. 2i ), which removed organic components. The survival of the NP superstructure can be rationalized based on the shrinkage of the gyroidal network. First, ~20% decrease of gyroidal node-to-node distance is observed in the structure after the plasma treatment (compare Fig. 2e with i ), accompanied with smaller NP–NP spacings in the struts. Furthermore, from high-angle annular dark-field imaging-STEM image analysis thinning of the gyroidal struts is evidenced (see Supplementary Fig. 3a,b ). Therefore, the plasma-treated NP network may move above the percolation threshold without organic materials, thus maintaining the superstructure. SCFT simulations We used a recently developed SCFT/density functional theory approach to incorporate molecular details of ligand-stabilized Pt NPs [16] , [17] . To observe NP distribution variations for a fixed morphology, a symmetry-adopted real space basis set for the space group Q 214 was used [17] . As a reference system, we chose one of the simulated systems discussed in Hur et al. [17] , where the predicted morphology is G A , interaction parameter between ligand and C block χ C,Ligand N= 0, N L =20 and NP volume fraction, ϕ P +ϕ Ligand =0.06 (note that, owing to similar χ parameters for PDMAEMA and polyethylene oxide [23] , [42] , simulation parameters for polyethylene oxide were used for the C block in this work). For Fig. 5e , two times longer ligands with N L =60 than those of the reference system were used. For Au NPs of Fig. 5j,k , the same parameters of Pt NPs in Fig. 4e were used but the number of ligands per NP and interaction parameter between B block and ligands were varied as N L =210 and χ B,Ligand N= 40. How to cite this article: Li, Z. et al. Linking experiment and theory for three-dimensional networked binary metal nanoparticles—triblock terpolymer superstructures. Nat. Commun. 5:3247 doi: 10.1038/ncomms4247 (2014).